Large-scale complementary macroelectronics using hybrid integration of carbon nanotubes and IGZO thin-film transistors Carbon nanotubes and metal oxide semiconductors have emerged as important materials for p-type and n-type thin-film transistors, respectively; however, realizing sophisticated macroelectronics operating in complementary mode has been challenging due to the difficulty in making n-type carbon nanotube transistors and p-type metal oxide transistors. Here we report a hybrid integration of p-type carbon nanotube and n-type indium–gallium–zinc-oxide thin-film transistors to achieve large-scale (>1,000 transistors for 501-stage ring oscillators) complementary macroelectronic circuits on both rigid and flexible substrates. This approach of hybrid integration allows us to combine the strength of p-type carbon nanotube and n-type indium–gallium–zinc-oxide thin-film transistors, and offers high device yield and low device variation. Based on this approach, we report the successful demonstration of various logic gates (inverter, NAND and NOR gates), ring oscillators (from 51 stages to 501 stages) and dynamic logic circuits (dynamic inverter, NAND and NOR gates). During the past few decades, many thin-film materials have emerged with great significance for the development of macroelectronics, such as organic semiconductors, oxide semiconductors (for example, indium–gallium–zinc oxide (IGZO)) and, more recently, carbon nanotubes (CNTs) [1] , [2] , [3] , [4] . Organic thin-film transistors (TFTs) have shown tremendous progress in terms of their effective device mobility, hence making them attractive candidates for the implementation of macroelectroincs [3] , [5] , [6] , [7] , [8] , [9] . However, the environmental and operational stability of organic TFTs still remains an important issue to be addressed for their usage in practical macroelectronic applications [3] , [5] , [9] , [10] . Oxide semiconductor TFTs such as IGZO-based TFTs have been successfully employed in pixel driver circuitry for commercial display applications [4] , [11] , [12] , [14] . Despite the advancement in oxide semiconductor TFT technology, oxide semiconductor thin films are usually n-type materials, and it still remains a challenge to produce stable p-type oxide TFTs with high effective TFT mobility for macroelectronics [4] , [15] , [16] . On the other hand, carbon nanotube network thin film has emerged as a potential building block for macroelectronics such as back-panel organic light-emitting diode pixel-driving circuits for active-matrix flat-panel displays [17] , [18] , digital circuits [19] , [20] , [21] , [22] , [23] , [24] , [25] , [26] , [27] , radio frequency identification tags [28] , sensors [29] , [30] , [31] and memories [32] . CNT network TFTs exhibit the merits of high transparency, high flexibility, low process cost, low processing temperature and high scalability, while traditional TFT materials such as amorphous silicon and polycrystalline silicon are usually not transparent, have poor flexibility, require high processing cost and use high processing temperature [20] , [23] , [33] , [34] , [35] , [36] , [37] , [38] , [39] . However, semiconducting CNTs are usually p-type semiconducting materials in atmosphere due to adsorption of oxygen [40] , [41] , [42] , and techniques to convert CNTs to n-type semiconductors [22] , [41] , [43] , [44] , [45] , [46] , [47] , [48] , [49] still require further development to achieve long-term stability (for example, over multiple years), and sometimes bear significant device-to-device variation [22] , [46] , [49] . It is clear that obtaining both p-type and n-type TFTs is of utmost importance in producing complementary macroelectronic circuits with minimal steady-state power dissipation, and doing so with high device yield and low device-to-device variation would be essential for large-scale integration of macroelectronics. Here, we report a hybrid integration of p-type CNT and n-type IGZO thin-film transistors to achieve large-scale (>1,000 transistors) complementary macroelectronic circuits on both rigid and flexible substrates. IGZO is selected to be expended as the channel material for the n-type transistors in our integrated macroelectronic circuits, owing to the fact that IGZO is one of the most promising members in the category of amorphous oxide semiconductors with desirable electrical performance [4] , [50] , [51] . This novel approach of hybrid integration allows us to combine the strength of CNT TFTs behaving as p-type devices and IGZO TFTs behaving as n-type devices, thus circumventing the difficulty of producing n-type CNT and p-type metal oxide TFTs. More importantly, this approach offers high device yield and low device variation, as manifested by the demonstration of various logic gates (inverter, NAND and NOR gates), ring oscillators (from 51 stages to 501 stages) and dynamic logic circuits (dynamic inverter, NAND and NOR gates), as discussed below. Hybrid complementary CNT and IGZO TFTs and circuits Schematic diagram in Fig. 1a illustrates our proposed scheme of a hybrid integration of CNT network and IGZO TFTs in an inverter, which can be fabricated on both of a rigid Si/SiO 2 and a flexible polyimide (PI) substrate. We have adopted an individual back-gate design for all of the circuits fabricated in this study, and detail description of the fabrication process can be found in the Methods section and in the Supplementary Fig. 1 . Briefly, individual back-gate Ti/Au electrodes were patterned and deposited on a Si/SiO 2 substrate. The process was followed by deposition of dielectric materials (40 nm of Al 2 O 3 and 5 nm of SiO x ), and incubation in poly- L -lysine solution for 6 min. The poly- L -lysine solution was then washed away with deionized (DI) water and dried with N 2 air gun, and a thin layer of poly- L -lysine was left behind on the sample to act as an adhesive layer for the nanotubes. The substrate was then incubated in 98% semiconducting nanotube solution and then was rinsed with DI water and dried with N 2 air gun, which left a uniform carbon network on the substrate. The 98% semiconducting CNT network solution was used as purchased from NanoIntegris, for which a density gradient ultracentrifugation approach was used to separate semiconducting and metallic nanotubes [20] , [33] , [52] . Metallization of Ti/Pd was carried out after patterning the CNT thin film for the specific channel geometry of the p-type TFTs. Then a layer of IGZO thin film was deposited as the channel material for the n-type devices by radio frequency magnetron sputtering. Finally, the circuit was completed by conducting standard photolithography and metallization of Ti/Au for the n-type TFTs. The schematic diagram in Fig. 1b conceptually illustrates the interface between the CNT random network and the Ti/Pd electrode. 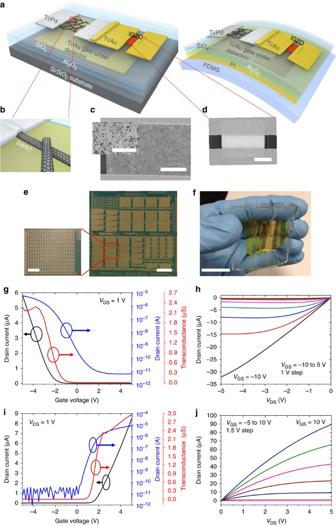Figure 1: Schematic diagrams, images and device characteristics of hybrid CNT/IGZO complementary integrated circuits. (a) Three-dimensional schematic diagram of a CNT/IGZO complementary mode inverter on rigid substrate (left) and same circuit on flexible substrate (right). (b) Schematic diagram conceptually showing the interface between the Ti/Pd electrode and the CNT network. (c) Scanning electron microscopic (SEM) image of CNT network in the channel of a p-type TFT; the scale bar in the low magnification SEM image is 10 μm and the scale bar in the high magnification SEM image is 2 μm. (d) SEM image of IGZO in an n-type TFT; scale bar, 5 μm. (e) Optical micrograph of the hybrid CNT/IGZO ring oscillators, inverters, individual p-type and n-type transistors fabricated on a rigid Si/SiO2substrate. The inset shows a 501-stage ring oscillator on the rigid substrate. The scale bar in the rigid circuit chip is 500 μm. The scale bar in the 501-stage ring oscillator image is 600 μm. (f) Optical photographic image of the hybrid CNT/IGZO ring oscillators, inverters and individual transistors on a flexible PI substrate laminated on a polydimethylsiloxane (PDMS) film. The scale bar in flexible circuit is 2 cm. (g) Transfer characteristic in linear and log scale and transconductance of a CNT TFT with gate bias varied from −5 to 5 V. Channel length (Lch)=20 μm, channel width (Wch)=100 μm, drain-source voltage (VDS)=1 V. (h) Output characteristic of the CNT TFT withVDSvaried from −5 to 0 V. (i) Transfer characteristic in linear and log scale and transconductance of a IGZO TFT with gate bias varied from −5 to 5 V.Lch=4 μm,Wch=12 μm,VDS=1 V. (j) Output characteristic of the IGZO TFT withVDSvaried from 0 to 5 V. Figure 1c,d shows scanning electron microscopic images illustrating the CNT network and IGZO thin film in the channel of p-type and n-type transistors, respectively. Figure 1e,f shows optical images of our hybrid-integrated CNT/IGZO complementary circuits on a rigid and a flexible substrate, including 501-stage ring oscillators, 251-stage ring oscillators, 101-stage ring oscillators, 51-stage ring oscillators, inverters and individual n-type and p-type devices. In addition to fabrication of the circuits on a rigid silicon/silicon oxide substrate, we successfully incorporated the integrated circuits onto a flexible PI membrane (HD MircroSystems, PI-2525). The result has provided evidence for the applicability of large-scale integration of flexible electronics using CNT TFTs. The detail of the fabrication procedure of CNT/IGZO hybrid circuits on flexible substrate can be found in Methods section and in the Supplementary Fig. 1 . The hybrid CNT/IGZO-integrated circuits were characterized for their electrical performance as described in later sections of this report. The details of the electrical characterizations can be found in the Methods section. Figure 1: Schematic diagrams, images and device characteristics of hybrid CNT/IGZO complementary integrated circuits. ( a ) Three-dimensional schematic diagram of a CNT/IGZO complementary mode inverter on rigid substrate (left) and same circuit on flexible substrate (right). ( b ) Schematic diagram conceptually showing the interface between the Ti/Pd electrode and the CNT network. ( c ) Scanning electron microscopic (SEM) image of CNT network in the channel of a p-type TFT; the scale bar in the low magnification SEM image is 10 μm and the scale bar in the high magnification SEM image is 2 μm. ( d ) SEM image of IGZO in an n-type TFT; scale bar, 5 μm. ( e ) Optical micrograph of the hybrid CNT/IGZO ring oscillators, inverters, individual p-type and n-type transistors fabricated on a rigid Si/SiO 2 substrate. The inset shows a 501-stage ring oscillator on the rigid substrate. The scale bar in the rigid circuit chip is 500 μm. The scale bar in the 501-stage ring oscillator image is 600 μm. ( f ) Optical photographic image of the hybrid CNT/IGZO ring oscillators, inverters and individual transistors on a flexible PI substrate laminated on a polydimethylsiloxane (PDMS) film. The scale bar in flexible circuit is 2 cm. ( g ) Transfer characteristic in linear and log scale and transconductance of a CNT TFT with gate bias varied from −5 to 5 V. Channel length ( L ch )=20 μm, channel width ( W ch )=100 μm, drain-source voltage ( V DS )=1 V. ( h ) Output characteristic of the CNT TFT with V DS varied from −5 to 0 V. ( i ) Transfer characteristic in linear and log scale and transconductance of a IGZO TFT with gate bias varied from −5 to 5 V. L ch =4 μm, W ch =12 μm, V DS =1 V. ( j ) Output characteristic of the IGZO TFT with V DS varied from 0 to 5 V. Full size image Based on the scanning electron microscopic image of the CNTs in the device channel ( Fig. 1c ), it illustrates a uniform network of CNTs. The metrics of performance of the p-type devices can be readily controlled by varying the density of the CNTs in the channel through modification of the CNT incubation time [20] . Figure 1g,h delineates the electrical performance of an individual p-type CNT TFT. The CNT TFT, as expected, exhibits a p-type transistor behaviour as shown in the transfer characteristic curve (black curve) of Fig. 1g . The device exhibits a desirable p-type transistor behaviour, the typical device current on/off ratio ( I on / I off ) and mobility are ~10 5 –10 6 and 8–15 cm 2 V −1 s −1 , respectively. In this device and the devices utilized in the more complicated integrated circuits in our study, the channel length and width of the p-type transistors are 20 μm and 100 μm, respectively. The mobility was calculated based on the formula, , where C was the gate capacitance estimated with the network model [46] . The transistor can be fully saturated as depicted in Fig. 1h . Figure 1i,j illustrates the transfer and output characteristic of an individual n-type IGZO TFT with a channel length of 4 μm and a channel width of 12 μm. The typical I on / I off and mobility of an n-type device are ~10 6 and ~7–8 cm 2 V −1 s −1 , respectively. Based on the results presented in Fig. 1g,i , the p-type and n-type devices turn on approximately at −2 V and 1.8 V, respectively. We measured the performance of 20 individual p-type CNT and n-type IGZO TFTs, and they exhibited relatively uniform results. Histograms of the mobility, current on/off ratio and threshold voltage of those devices are shown in Fig. 2 . Circuits operating in complementary mode can be actualized with the desirable p-type and n-type behaviour of these TFTs. CNT and IGZO TFT are an ideal pair of materials for complementary integrated circuits. The fabrication process of the devices based on the two materials can be conducted at room temperature, which is compatible with the current flat-panel display manufacturing processes, and it is also desirable for flexible electronics. 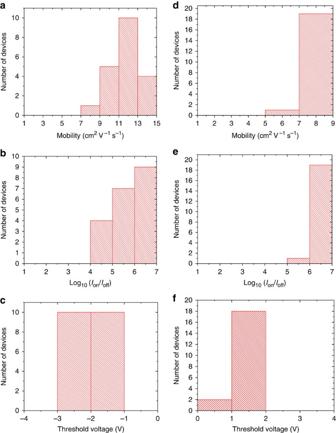Figure 2: Histograms of mobility, current on/off ratio and threshold voltage of 20 CNT-based and 20 IGZO-based TFTs. (a) Histogram of mobility of 20 CNT devices fabricated on a rigid substrate showing an average mobility of 11.8 cm2V−1s−1with 10 of the devices showing mobility between 11 and 13 cm2V−1s−1. (b) Histogram of current on/off ratio (log10(Ion/Ioff)) measured from the same 20 devices with 16 devices showingIon/Ioffbetween 1 × 105and 1 × 107. (c) Histogram of the threshold voltage (Vth) measured from the 20 CNT TFTs, showing the meanVthto be −2.2 V, and all of the devices showingVthbetween −3 and −1 V. (d) Histogram of mobility exhibited by the 20 IGZO devices fabricated on a rigid substrate, having an average mobility of 7.9 cm2V−1s−1, and 19 of the devices showing mobility between 7 and 9 cm2V−1s−1. (e) Histogram of log10(Ion/off) measured from the same 20 devices with 19 devices showing current on/off ratio between 1 × 106and 1 × 107. (f) Histogram ofVthmeasured from the 20 IGZO TFTs having the meanVthbeing 1.2 V, and 18 of the devices showingVthbetween 1 and 2 V. Figure 2: Histograms of mobility, current on/off ratio and threshold voltage of 20 CNT-based and 20 IGZO-based TFTs. ( a ) Histogram of mobility of 20 CNT devices fabricated on a rigid substrate showing an average mobility of 11.8 cm 2 V −1 s −1 with 10 of the devices showing mobility between 11 and 13 cm 2 V −1 s −1 . ( b ) Histogram of current on/off ratio (log 10 ( I on / I off )) measured from the same 20 devices with 16 devices showing I on / I off between 1 × 10 5 and 1 × 10 7 . ( c ) Histogram of the threshold voltage ( V th ) measured from the 20 CNT TFTs, showing the mean V th to be −2.2 V, and all of the devices showing V th between −3 and −1 V. ( d ) Histogram of mobility exhibited by the 20 IGZO devices fabricated on a rigid substrate, having an average mobility of 7.9 cm 2 V −1 s −1 , and 19 of the devices showing mobility between 7 and 9 cm 2 V −1 s −1 . ( e ) Histogram of log 10 ( I on/off ) measured from the same 20 devices with 19 devices showing current on/off ratio between 1 × 10 6 and 1 × 10 7 . 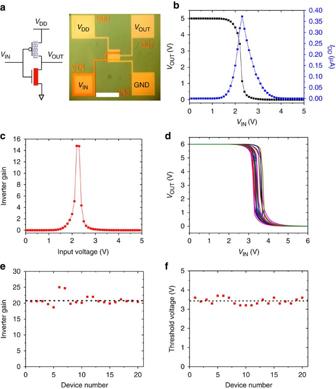Figure 3: Schematic diagram, optical micrograph and characteristic of a hybrid CNT/IGZO complementary inverter. (a) Schematic diagram and an optical micrograph of a hybrid CNT/IGZO inverter fabricated on a rigid Si/SiO2substrate. Scale bar, 200 μm.VDDis designated as the supplied voltage of the circuits.VOUTcorresponds to the output signal of the circuits.VINcorresponds to the input signal of the inverter and GND is designated as the ground of the circuits. (b) Output voltage and current characteristic of the hybrid inverter. (c) Voltage gain of the inverter. (d) Output characteristic of 20 hybrid CNT/IGZO inverters fabricated on a PI flexible substrate. (e) Voltage gain of the 20 inverters with a mean value of 20.9 and a s.d. of 1.5. (f) Threshold voltage (atVout=Vin) of the 20 inverters with a mean value of 3.4 V and a s.d. of 0.17 V. ( f ) Histogram of V th measured from the 20 IGZO TFTs having the mean V th being 1.2 V, and 18 of the devices showing V th between 1 and 2 V. Full size image Hybrid CNT/IGZO inverter on rigid and flexible substrates Figure 3 describes the operation of hybrid inverters ( Fig. 3a–c from rigid substrate, Fig. 3d–f from flexible substrate). Figure 3a demonstrates schematic diagram and an optical micrograph of a hybrid inverter fabricated on a Si/SiO 2 substrate. The supply voltage ( V DD ) and the ground (GND) of the inverter were connected to 5 and 0 V during the characterization. The inverter exhibits an ideal rail-to-rail output voltage behaviour as can be seen in Fig. 3b , and the inverter threshold voltage is measured to be at 2.4 V, which is nearly half of the V DD . The inverter current was around 190 pA when the input bias was below 1 V or above 4 V, hence demonstrating the low steady-state power dissipation advantage of having this hybrid complementary TFT structure. The inverter exhibits a voltage gain of 15 as shown in Fig. 3c . Figure 3d illustrates the uniformity of the performance of 20 hybrid CNT/IGZO inverters fabricated on flexible PI substrate. The 20 inverters were measured in the same region of the chip, and the yield of the circuits is 100%. This demonstrates the high yield and practicality of implementing this hybrid circuit scheme for both rigid and flexible circuit applications. The uniformity of the performance of the 20 inverters in terms of their voltage gain and threshold voltage is shown in Fig. 3e,f . Figure 3: Schematic diagram, optical micrograph and characteristic of a hybrid CNT/IGZO complementary inverter. ( a ) Schematic diagram and an optical micrograph of a hybrid CNT/IGZO inverter fabricated on a rigid Si/SiO 2 substrate. Scale bar, 200 μm. V DD is designated as the supplied voltage of the circuits. V OUT corresponds to the output signal of the circuits. V IN corresponds to the input signal of the inverter and GND is designated as the ground of the circuits. ( b ) Output voltage and current characteristic of the hybrid inverter. ( c ) Voltage gain of the inverter. ( d ) Output characteristic of 20 hybrid CNT/IGZO inverters fabricated on a PI flexible substrate. ( e ) Voltage gain of the 20 inverters with a mean value of 20.9 and a s.d. of 1.5. ( f ) Threshold voltage (at V out = V in ) of the 20 inverters with a mean value of 3.4 V and a s.d. 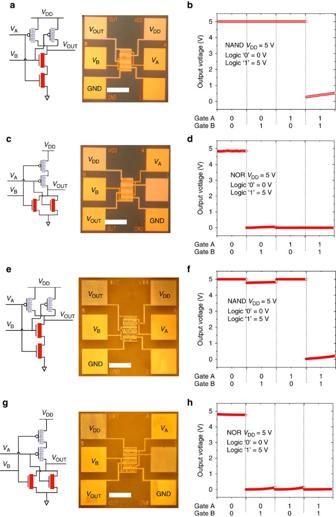Figure 4: Schematic diagrams, optical micrographs and output characteristic of complementary hybrid NAND and NOR logic gates on rigid Si/SiO2substrate (a–d), and on flexible PI substrate (e–h). (a) Schematic diagram and optical micrograph of a hybrid CNT/IGZO NAND gate on a rigid substrate. Scale bar, 200 μm.VAandVBare used to designate the two input signals of circuits.VDD,VOUTand GND correspond to the supplied voltage, the output signal and the ground of the NAND gate, respectively. Same denotation of the labels is applied to the schematic of the NOR gate. A supplied voltage of 5 V was supplied to the circuit during measurement. Input signals of ‘00’, ‘01’, ‘10’ and ‘11’ were supplied to the logic gate. (b) Output characteristic of the hybrid CNT/IGZO NAND gate. (c) Schematic diagram and optical micrograph of a hybrid CNT/IGZO NOR gate on a rigid substrate. Scale bar, 200 μm. (d) Output characteristic of the hybrid CNT/IGZO NOR gate. (e) Schematic diagram and optical micrograph of a hybrid NAND gate fabricated on a PI substrate. The scale bar in the optical micrograph is 200 μm. (f) Output characteristic of the hybrid NAND gate. (g) Schematic diagram and optical micrograph of a hybrid NOR gate fabricated on a PI substrate. The scale bar in the optical micrograph is 200 μm. (h) Output characteristic of the hybrid NOR gate. of 0.17 V. Full size image CNT/IGZO NAND and NOR gates on rigid and flexible substrates Figure 4a–d illustrates the performance of a two-input NAND gate and a two-input NOR gate fabricated based on the CNT/IGZO hybrid design on rigid substrates. Both of the NAND gate and NOR gate demonstrate a rail-to-rail voltage swing from 0 to 5 V at a supply voltage of 5 V. This can be attributed to the robust complementary mode of operation of the CNT/IGZO hybrid design. Figure 4b shows the output of the NAND gate returning correctly a signal ‘0’ only when both of the inputs are ‘1’. In that logic configuration, both of the p-type CNT transistors are turned off. Figure 4d illustrates the output of the NOR gate returning correctly an output of ‘1’ only at the condition when both of the inputs are set to ‘0’. This logic corresponds to both of the n-type IGZO transistors are turned off. The circuits return correct output signal based on the corresponding input logics. NAND and NOR gates are some of the basic building blocks in modern digital integrated circuits. This enables us to further explore the possibility of more complex digital circuits with the hybrid circuit design. Figure 4e–h illustrates the performance of a CNT/IGZO hybrid-integrated two-input NAND and a two-input NOR gate fabricated on a flexible PI thin film, and the supply voltage of the two logic circuits is also 5 V. The output signal of the two logic gates demonstrate that the CNT/IGZO hybrid-integrated circuits returned correct logic output signals based on the corresponding input logics while operating on flexible substrates. This further demonstrates the potential of implementing the hybrid CNT/IGZO circuit configuration for circuits built on both rigid and flexible substrates. Figure 4: Schematic diagrams, optical micrographs and output characteristic of complementary hybrid NAND and NOR logic gates on rigid Si/SiO 2 substrate ( a – d ), and on flexible PI substrate ( e – h ). ( a ) Schematic diagram and optical micrograph of a hybrid CNT/IGZO NAND gate on a rigid substrate. Scale bar, 200 μm. V A and V B are used to designate the two input signals of circuits. V DD , V OUT and GND correspond to the supplied voltage, the output signal and the ground of the NAND gate, respectively. Same denotation of the labels is applied to the schematic of the NOR gate. A supplied voltage of 5 V was supplied to the circuit during measurement. Input signals of ‘00’, ‘01’, ‘10’ and ‘11’ were supplied to the logic gate. ( b ) Output characteristic of the hybrid CNT/IGZO NAND gate. ( c ) Schematic diagram and optical micrograph of a hybrid CNT/IGZO NOR gate on a rigid substrate. Scale bar, 200 μm. ( d ) Output characteristic of the hybrid CNT/IGZO NOR gate. ( e ) Schematic diagram and optical micrograph of a hybrid NAND gate fabricated on a PI substrate. The scale bar in the optical micrograph is 200 μm. ( f ) Output characteristic of the hybrid NAND gate. ( g ) Schematic diagram and optical micrograph of a hybrid NOR gate fabricated on a PI substrate. The scale bar in the optical micrograph is 200 μm. ( h ) Output characteristic of the hybrid NOR gate. 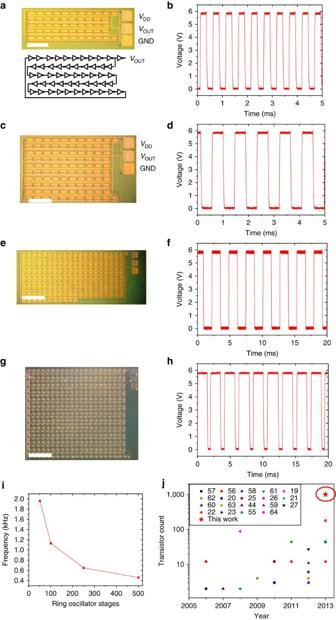Figure 5: Structure and output characteristic of 51-stage, 101-stage, 251-stage and 501-stage ring oscillators. (a) Optical micrograph and schematic diagram of a 51-stage ring oscillator. Scale bar, 400 μm. (b) Output characteristic of a 51-stage ring oscillator. (c,d) Optical micrograph of a 101-stage ring oscillator and its output characteristic, respectively. Scale bar, 400 μm. (e,f) Optical micrograph of a 251-stage ring oscillator and its output characteristic, respectively. Scale bar, 600 μm. (g,h) Optical micrograph of a 501-stage ring oscillator and its output characteristic, respectively. Scale bar, 600 μm. (i) Frequency of the output signals of the 51-stage, 101-stage, 251-stage and 501-stage ring oscillators with respect to the number of stages. (j) Comparison of the level of integration of CNT-based integrated circuits from 19 published articles and our work. The star circled by red ink corresponds to our work. Full size image Hybrid CNT/IGZO-integrated ring oscillators with 1,004 transistors Figure 5 describes the operation of 51-stage, 101-stage, 251-stage and 501-stage ring oscillators on rigid substrate. With the ideal inverter behaviour manifested by the hybrid CNT/IGZO-integrated circuit, the hybrid design enables implementation of 51-stage, 101-stage, 251-stage and 501-stage ring oscillators, and they all generated output signals with rail-to-rail output voltage swing from 0 to 6 V. The optical micrographs and output signals of the oscillators are depicted in Fig. 5a–h . The schematic diagram in Fig. 5a , illustrates the circuit connection of a 51-stage ring oscillator. The labels V DD , V OUT and GND correspond to the supplied voltage, the output voltage and the ground for the ring oscillators, respectively. In the oscillator, 51 hybrid CNT/IGZO complementary inverters are connected in series with an additional inverter connected at the output of the oscillator functioning as a buffer stage. The circuit configuration is adopted for all of the oscillators presented in this work. The oscillation frequency of ring oscillators decreases with increase in number of stages due to the effect of stage delay. This effect is depicted in Fig. 5i , showing the oscillation frequencies at 1.96 kHz, 1.13 kHz, 648 Hz and 460 Hz for 51-stage, 101-stage, 251-stage and 501-stage ring oscillator, respectively. All of the results were obtained from the circuits fabricated on one single chip, which underscores the robustness of hybrid CNT/IGZO design. The stage delay of the 51-stage ring oscillator can be calculated with 1/2 nf , n being the number of stages in an oscillator, and f being the oscillation frequency. The stage delay is found to be 5 μs, which is consistent for all the oscillators studied in this report. We note that our ring oscillator performance compares favourably with previously published work [23] . For instance, all of our ring oscillators exhibited rail-to-rail switching between V DD and ground. In comparison, previous work based on p-type-only inverters showed oscillation that reached neither V DD nor ground [23] . Figure 5: Structure and output characteristic of 51-stage, 101-stage, 251-stage and 501-stage ring oscillators. ( a ) Optical micrograph and schematic diagram of a 51-stage ring oscillator. Scale bar, 400 μm. ( b ) Output characteristic of a 51-stage ring oscillator. ( c , d ) Optical micrograph of a 101-stage ring oscillator and its output characteristic, respectively. Scale bar, 400 μm. ( e , f ) Optical micrograph of a 251-stage ring oscillator and its output characteristic, respectively. Scale bar, 600 μm. ( g , h ) Optical micrograph of a 501-stage ring oscillator and its output characteristic, respectively. Scale bar, 600 μm. ( i ) Frequency of the output signals of the 51-stage, 101-stage, 251-stage and 501-stage ring oscillators with respect to the number of stages. ( j ) Comparison of the level of integration of CNT-based integrated circuits from 19 published articles and our work. The star circled by red ink corresponds to our work. Full size image We were able to demonstrate the largest integration of hybrid CNT/IGZO circuit with a 501-stage ring oscillator, which was comprised of 1,004 transistors as illustrated in the optical image in Fig. 5g . This large-scale integrated circuit is consisted of 501 inverters and a buffer stage. The V DD of the circuit is 6 V, and as can be observed in Fig. 5h , the output of the oscillator is showing a rail-to-rail voltage swing. The oscillation frequency of the circuit can reach 460 Hz, which is a result of combination of the stage delay across the circuit. All of the aforementioned measurements were taken in ambient environment, indicating the stability of the CNT and IGZO transistors. After stored in air for 1 week, IGZO transistors did show reduction in on-state current by ~30%, which could be attributed to the interaction between IGZO thin film and oxygen and moisture in air [4] , [53] , [54] . However, the deterioration on the electrical performance of the IGZO TFTs saturated, as on-state current of the same IGZO TFT measured 1 year after its first characterization maintained at a level that is ~50% less than its first characterized value, that is, from ~10 μA to ~5 μA. CNT transistors exhibited little degradation. After being stored in vacuum for 1 month, the 51-stage ring oscillator still operated correctly, however, with deteriorated output amplitude. Further passivation of the samples using dielectric material coating (for example, Al 2 O 3 ) should alleviate or eliminate the effect of degradation of the IGZO TFTs [53] , [54] . The CNT/IGZO hybrid circuit platform provides a high-yield foundation for the integration with such unprecedented level of integration. Figure 5j delineates the progress of the level of integration of carbon nanotube-based circuits since the year 2006, including the result from our study and data reported by other research teams [19] , [20] , [21] , [22] , [23] , [25] , [26] , [27] , [44] , [55] , [56] , [57] , [58] , [59] , [60] , [61] , [62] , [63] , [64] . A general trend of increment in the level of integration can be observed on the graph, and we have realized the first demonstration of large-scale integrated circuits based on hybrid integration of 502 CNT transistors and 502 IGZO transistors. 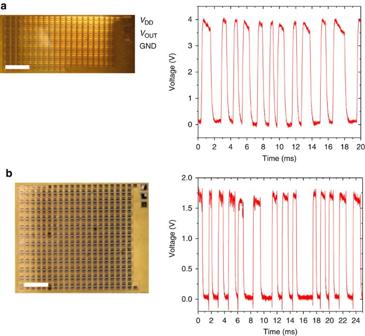Figure 6: Optical micrograph and output characteristic of a hybrid 251-stage ring oscillator and a hybrid 501-stage ring oscillator fabricated on flexible PI substrate. (a) Optical micrograph and output characteristic of a 251-stage hybrid complementary ring oscillator fabricated on a flexible PI substrate. The oscillation frequency was 338 Hz and output signal oscillated between 0 and 4 V, and the supplied voltage was 6 V. (b) Optical micrograph and output characteristic of a 501-stage hybrid complementary ring oscillator fabricated on a flexible PI substrate. The oscillation frequency was 294 Hz and the output signal oscillated between 0 and 1.8 V, and the supplied voltage was 6 V. Figure 6a,b demonstrates a hybrid CNT/IGZO 251-stage and a 501-stage ring oscillator fabricated on flexible PI films, and their corresponding output characteristics. Figure 6: Optical micrograph and output characteristic of a hybrid 251-stage ring oscillator and a hybrid 501-stage ring oscillator fabricated on flexible PI substrate. ( a ) Optical micrograph and output characteristic of a 251-stage hybrid complementary ring oscillator fabricated on a flexible PI substrate. The oscillation frequency was 338 Hz and output signal oscillated between 0 and 4 V, and the supplied voltage was 6 V. ( b ) Optical micrograph and output characteristic of a 501-stage hybrid complementary ring oscillator fabricated on a flexible PI substrate. The oscillation frequency was 294 Hz and the output signal oscillated between 0 and 1.8 V, and the supplied voltage was 6 V. Full size image Hybrid CNT/IGZO dynamic circuits In addition to the static logic gates and ring oscillators, we also demonstrate the implementation of dynamic logic circuits with the CNT/IGZO hybrid scheme. Dynamic logic gates are defined as the following [65] : ‘the operation of all dynamic logic gates depends on temporary (transient) storage of charge in parasitic node capacitances, instead of relying on steady-state circuit behaviour.’ The advantage of dynamic logic gate is that it increases the overall switching speed of the circuits and reduces static power dissipation comparing with static logic circuits. 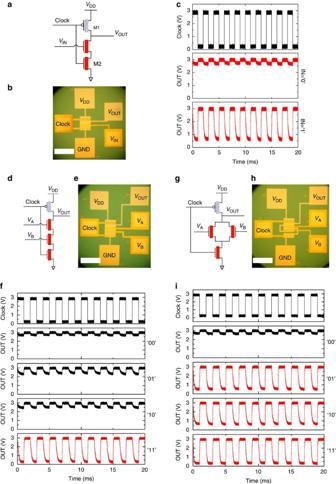Figure 7: Structure and output characteristic of dynamic inverter, NAND and NOR gate. (a,b) Schematic and optical micrograph of a dynamic inverter based on the hybrid CNT/IGZO complementary scheme. Scale bar, 200 μm. (c) Output characteristic of the dynamic inverter with a clock signal supplied at 500 Hz and aVDDof 3 V. (d,e) Schematic and optical micrograph of a dynamic NAND gate. Scale bar, 200 μm. (f) Output characteristic of the dynamic NAND gate with a clock signal supplied at 500 Hz and aVDDof 3 V. (g,h) Schematic and optical micrograph of a dynamic NOR gate. Scale bar, 200 μm. (i) Output characteristic of the dynamic NOR gate with a clock signal supplied at 500 Hz and aVDDof 3 V. Figure 7a–c illustrates the performance of a dynamic inverter. In a dynamic inverter, a clock signal is sent into the circuit. When the clock signal is low, M1 is turned on to precharge the output parasitic capacitance to the level of V DD , and M2 is off during this cycle of operation, and hence the input cannot affect the output when the clock signal is low. When the clock signal is changed to high, M1 is turned off and now M2 is on, at which the output is determined by the input signal, and this is the evaluating stage. To the best of our knowledge, our report is the first demonstration of using CNT in a dynamic gate-integrated circuit. The V DD of the inverter was held at 3 V in the middle panel of Fig. 7c , and the clock signal was set at 500 Hz as depicted in the upper panel of the same figure. The middle panel and the lower panel of Fig. 7c illustrate the output signal versus time for the input signal of ‘0’ and ‘1’, respectively. As we can see from both of the panels, when clock is low, the output is ‘1’ (near V DD ) regardless of the input. When the clock is high, the output is an inverted signal of the input, as expected. Equivalently, the output of the inverter was observed to be near V DD when the input was ‘0’ ( Fig. 7c middle panel), and the output resulted in an inverted signal of the clock when the input was set at ‘1’ (3 V) (in the lower panel of the figure). Figure 7: Structure and output characteristic of dynamic inverter, NAND and NOR gate. ( a , b ) Schematic and optical micrograph of a dynamic inverter based on the hybrid CNT/IGZO complementary scheme. Scale bar, 200 μm. ( c ) Output characteristic of the dynamic inverter with a clock signal supplied at 500 Hz and a V DD of 3 V. ( d , e ) Schematic and optical micrograph of a dynamic NAND gate. Scale bar, 200 μm. ( f ) Output characteristic of the dynamic NAND gate with a clock signal supplied at 500 Hz and a V DD of 3 V. ( g , h ) Schematic and optical micrograph of a dynamic NOR gate. Scale bar, 200 μm. ( i ) Output characteristic of the dynamic NOR gate with a clock signal supplied at 500 Hz and a V DD of 3 V. Full size image Figure 7d–f shows the circuit and output characteristic of a dynamic NAND gate with a 3-V V DD . It generates correct output corresponding to the specific input signals as illustrated in Fig. 7f , the output is held near the V DD while the input signals are ‘00’, ‘01’ and ‘10’. The output returns an inverted signal of the clock when the input equals ‘11’. A dynamic NOR gate and its output characteristic are exemplified in Fig. 7g–i . The correct output signal close to V DD was generated by the dynamic gate when ‘00’ was supplied to the input ( Fig. 7i ). The output resulted in an inverted signal of the clock when ‘01’, ‘10’ and ‘11’ were supplied to the input of the NOR gate. This is the first demonstration of CNT-based dynamic inverter, NAND and NOR gates. It provides evidence that our hybrid circuit scheme can enable the integration of more complicated circuits with the dynamic circuit-building blocks. We have demonstrated with our experimental results that the carbon nanotube and IGZO hybrid complementary TFTs can be used as building blocks to realize large-scale integrated digital circuits with >1,000 transistors. Having the circuits operated in complementary mode can minimize the static-state power dissipation in the circuits. The p-type CNT TFT transistors are based on semiconducting enriched CNT solution, the performance of the transistors can be further improved by utilizing CNT solution with higher semiconducting purity. We have also demonstrated the operation of the circuits on a flexible PI substrate and the high yield of the devices on the substrate. This demonstration allows further development in the implementation of the hybrid CNT/IGZO circuit scheme for flexible electronics. Currently, the IGZO thin film employed in our circuits were fabricated with the sputtering technique; however, the material can also be printed during the fabrication procedure [66] . CNT thin film has also been demonstrated to exhibit desirable printability and performance for printed electronics [67] . For future development, the hybrid CNT/IGZO complementary circuit configuration can be investigated for large scale and low-cost printed electronics applications. Our approach of hybrid integration of p-type nanomaterial, in this case CNT and n-type oxide semiconductor, in this study, IGZO thin-film transistors, can have great impact on various macroelectronic applications. Fabrication of hybrid CNT/IGZO TFTs and integrated circuits Individual bottom-gate electrodes were patterned by photolithography on a highly doped p-Si substrate with a layer of thermally grown oxide (300 nm). E-beam evaporation was used to deposit Ti/Au (5 nm/50 nm) to form the electrodes. A layer of 40 nm of Al 2 O 3 was deposited on the electrodes by atomic layer deposition at 250 °C, which was then followed by deposition of 5 nm of SiO x by E-beam evaporation to form the dielectric layer for the circuits. In order to deposit carbon nanotube onto the dielectric material, the sample was functionalized by poly- L -lysine (0.1% wt in water from Ted Pella) to form amine-terminated surface. The surface of the dielectric material was covered with poly- L -lysine by drop-casting of the solution, and the surface was incubated in the solution for 6 min. Then, the sample was cleansed by DI water to remove the solution. Next, the solution of 0.01 mg ml −1 98% semiconducting CNTs (NanoIntegris) was dispensed from a micropipette by dropping to fully cover the surface of the functionalized sample. The sample with the dropped solution was left in air for 10 min, and then rinsed with DI water and dried with N 2 gun. CNT channels were then defined by photolithography and followed by O 2 plasma etching at 100 W/150 mTorr for 1 min and 15 s. Vias or interconnects between devices and probing window on testing pads for gate electrodes were patterned by photolithography, and the dielectric material at the vias and on the testing pads was etched by buffered oxide etchant (buffered HF 7:1) for 1 min and 20 s. Then, electrodes for the p-type CNT TFTs were defined by photolithography and then formed by E-beam evaporation with Ti/Pd (1 nm/50 nm). The IGZO channels were defined by standard photolithography. Then, 50 nm of IGZO thin film was deposited by radio frequency magnetron sputtering at 180 W. Finally the circuits were completed by patterning the electrodes for the n-type IGZO TFTs and metallization of Ti/Au (1 nm/50 nm) with E-beam evaporator. The fabrication of the CNT/IGZO hybrid complementary circuits can be conducted on flexible PI substrate with the procedure similar to the aforementioned steps. The only difference is that, initially a layer of PI (HD MicroSystems, PI-2525) was spun on the silicon-supporting wafer at a speed of 2,000 r.p.m. for 30 s. Then it was soft baked at 120 °C for 30 s, and then at 150 °C for 30 s. The second layer of PI was spun onto the sample and baked at the same conditions. Then the sample was cured in argon gas at a temperature of 200 °C for 30 min with a ramping rate of 4 °C per min. Then the temperature was raised to 300 °C at a ramping rate of 2.5 °C per min., and the temperature was sustained at the same level for 60 min. The thickness of the final PI film is approximately 24 μm. The circuits were then fabricated onto the PI substrate based on the procedure described in the previous paragraph. The fully fabricated circuits along with the PI film were delaminated from the Si/SiO 2 substrate, and were then laminated onto a polydimethylsiloxane substrate as a support to form a flexible IC chip. Characterization of hybrid CNT/IGZO TFTs and integrated circuits Characterization of individual CNT and IGZO TFT, as well as static hybrid CNT/IGZO inverter, NAND and NOR logic gates were conducted with an Agilent 4156B Precision Semiconductor Parameter Analyzer under ambient environment. The ring oscillators were characterized by supplying V DD and ground to the circuits through a DC power source (HP 6632A System DC Power Supply), and the output signals were measured with an oscilloscope (Agilent Infiniium MSO8104A). Measurements were performed on the dynamic inverter, NAND and NOR logic circuits with combined usage of the Semiconductor Parameter Analyzer and the oscilloscope. Input signals were supplied to the circuits with the Analyzer and the output signals were recorded with the oscilloscope. The flexible circuits were characterized with the same instruments as their rigid circuits counterparts. How to cite this article: Chen, H. et al . Large-scale complementary macroelectronics using hybrid integration of carbon nanotubes and IGZO thin-film transistors. Nat. Commun. 5:4097 doi: 10.1038/ncomms5097 (2014).